Enantioselective control of lattice and shape chirality in inorganic nanostructures using chiral biomolecules A large number of inorganic materials form crystals with chiral symmetry groups. Enantioselectively synthesizing nanostructures of such materials should lead to interesting optical activity effects. Here we report the synthesis of colloidal tellurium and selenium nanostructures using thiolated chiral biomolecules. The synthesis conditions are tuned to obtain tellurium nanostructures with chiral shapes and large optical activity. These nanostructures exhibit visible optical and chiroptical responses that shift with size and are successfully simulated by an electromagnetic model. The model shows that they behave as chiral optical resonators. The chiral tellurium nanostructures are transformed into chiral gold and silver telluride nanostructures with very large chiroptical activity, demonstrating a simple colloidal chemistry path to chiral plasmonic and semiconductor metamaterials. These materials are natural candidates for studies related to interactions of chiral (bio)molecules with chiral inorganic surfaces, with relevance to asymmetric catalysis, chiral crystallization and the evolution of homochirality in biomolecules. Chirality is the geometric property of structures that are non-superimposable with their mirror images. This characteristic is a fundamental aspect of biomolecules such as proteins and nucleic acids, rendering specificity in biomolecular recognition and structure–function relations. Although chiral crystals were considered as sources for the generation of homochirlity in biomolecules [1] , [2] , the opposite effect of biomolecules inducing homochirality in chiral crystals was not thoroughly addressed. Chiral systems also show unique optical (chiroptical) effects when interacting with polarized electromagnetic radiation. The effect commonly measured is circular dichroism (CD), the differential absorption of left and right circularly polarized light by chiral molecules and materials [3] . Unlike organic molecules, where the chiroptical effects are typically small at visible wavelengths, larger inorganic systems (roughly over ten nanometres to several hundreds of nanometres) may show stronger chiroptical effects [4] , [5] , [6] . Several mechanisms were suggested for induction of chiroptical phenomena in such systems (both metallic and semiconducting). In plasmonic nanosystems the dipolar near-field interaction [7] , or a far-field electromagnetic coupling [8] , [9] between a metal nanoparticle and a chiral molecule could lead to induction of CD in the plasmon resonance as well as enhancement of the molecular CD by the near-field coupling [10] , [11] . These effects, which may be useful for biomolecular sensing [9] , [12] and are fundamentally interesting, are nevertheless limited in magnitude. Stronger effects could be obtained in systems of achiral nanoparticles arranged in a chiral superstructure with strong interparticle interaction [13] , [14] , [15] , [16] . Recently, Kotov and colleagues [17] demonstrated that the chiroptical activity of a chiral particle dimer is intense enough to monitor on a single nanoparticle level. The most intuitive approach to obtain large chiroptical activity is by forming nanoparticles with an actual chiral shape such as a gammadion or a helix. This has been achieved by lithographic methods [18] , [19] , [20] . Recently, there have been several reports on the preparation of chiral inorganic nanostructures through non-lithographic methods: Liedl and colleagues [21] formed chiral plasmonic shapes using DNA Origami. Fischer and colleagues [22] used a unique setup for vapour deposition of inorganic materials with excellent control over shape, chirality and material composition. Kotov and colleagues [23] formed chiral metal nanoshells on initially achiral ZnO nanopillars by vacuum deposition at varying angles. Reports on formation of chiral shapes with enantiomeric excess for semiconductor [24] and mesoporous [25] , [26] materials also exist. In all these demonstrations the lattice symmetry of the crystal remains achiral and optical activity is obtained through the shape of the whole nanostructure. Many inorganic materials crystallize with a chiral lattice symmetry, and enantioselective nucleation and growth chemistry could be used to obtain non-racemic mixtures of nanocrystals of these materials. Saeva et al . [27] synthesized micron-scale selenium (Se) crystals in a chiral cellulose matrix. Trigonal Se (as well as tellurium (Te)) crystallizes in the chiral space group P 3 1 21 (or its enantiomorph P 3 2 21). In ref. 27 , the authors managed to get a sample with an enantiomeric excess of Se crystallites and measure CD at the electronic transitions of Se, but without structural characterization. The chiroptical activity was attributed to the lattice chirality of the crystals. The CD measurements in that work were probably strongly affected by light scattering and possible birefringence of the polymer matrix holding the Se microstructures. At the nanoscale, the concept was first demonstrated by us for cinnabar (α-HgS) nanocrystals that crystallize in the same chiral space group as Se and Te [28] . In that work, both enantiomers could be obtained, but the demonstration was still limited to lattice chirality only, and the obtained nanocrystal shape was achiral. In the present work, chiral nanocrystals of Te and Se with a variety of shapes, which exhibit chiroptical activity, are obtained. Previous reports on the synthesis of Te and Se nanomaterials [29] , [30] , [31] did not relate to the chirality or chiroptical activity of the nanostructures, and there were no attempts to direct their handedness. Here, in addition to lattice chirality of nanocrystals, the overall shape of Te nanocrystals is made chiral, to achieve a new level of control over chirality. Consequently, chirality can be controlled at two hierarchies, atomic lattice and mesoscale shape. These nanocrystals grow by a unique self-assembly process. A model simulation shows that the dominant chiroptical activity of these Te nanostructures comes from the shape chirality, rather than the chiral atomic arrangement. Furthermore, the reactivity of Te towards various chemical transformation processes allows templating other materials into chiral shapes. Synthesis of the Te and Se nanostructures Te and Se precursors were reduced in the presence of a large concentration of thiolated chiral biomolecules such as cysteine, penicillamine and glutathione, where the thiol group strongly binds to Te or Se. These biomolecules proved to be very efficient reducing agents through the thiol group oxidation, as previously discussed for the case of Te(IV) species [32] , [33] . An additional reducing agent, hydrazine, was added, in some cases, immediately before or after the fast reduction by the biomolecule. Shape control was achieved by varying the type of biomolecule used, order of reagent addition, reaction time and temperature. All the different samples obtained are depicted in the transmission electron microscopy (TEM) images in Fig. 1 (Te samples Fig. 1a–e and Se Fig. 1f , see also Supplementary Fig. 1 ). For all the samples, high-resolution TEM images and electron diffraction patterns verified the formation of the chiral trigonal crystal phase of these materials (see Supplementary Figs 2–5 ). All the syntheses were highly reproducible and repeated procedures for each sample always resulted in the same shape of particles and same CD spectra. In particular, the synthesis of the most intriguing sample 5 was repeated about 50 times reproducibly. 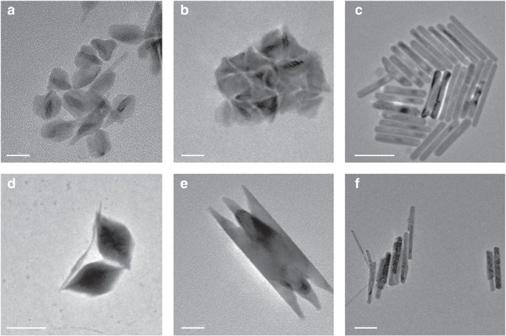Figure 1: TEM images of tellurium and selenium nanocrystals produced by different procedures. (a,b) Tellurium nanocrystals (sample 1), obtained with glutathione without hydrazine. Scale bar, 20 nm. Inb, the nanocrystals are packed closely, and aligned with their long axis perpendicular to the surface, exhibiting the trigonally symmetric cross section. (c) Long tellurium nanorods (sample 2), obtained with glutathione and hydrazine. Scale bar, 100 nm. (d) Tellurium nanocrystals (samples 3–4) obtained withL- orD-penicillamine and hydrazine. Scale bar, 200 nm. (e) Tellurium nanocrystal (sample 5), obtained with hydrazine and glutathione added in a reversed order of sample 2. Scale bar, 20 nm. (f) Selenium nanocrystals obtained with cysteine. Scale bar, 200 nm. Figure 1: TEM images of tellurium and selenium nanocrystals produced by different procedures. ( a , b ) Tellurium nanocrystals (sample 1), obtained with glutathione without hydrazine. Scale bar, 20 nm. In b , the nanocrystals are packed closely, and aligned with their long axis perpendicular to the surface, exhibiting the trigonally symmetric cross section. ( c ) Long tellurium nanorods (sample 2), obtained with glutathione and hydrazine. Scale bar, 100 nm. ( d ) Tellurium nanocrystals (samples 3–4) obtained with L - or D -penicillamine and hydrazine. Scale bar, 200 nm. ( e ) Tellurium nanocrystal (sample 5), obtained with hydrazine and glutathione added in a reversed order of sample 2. Scale bar, 20 nm. ( f ) Selenium nanocrystals obtained with cysteine. Scale bar, 200 nm. Full size image The difference in product shape/size on using different biomolecules might be attributed to the exact nature of reduction of cationic Te species by thiolates. As the Te reduction mechanism proceeds through initial formation of a complex of Te(IV) with four thiolate molecules [32] , the kinetics of the reaction should depend on the structure of the ligand molecule, which affects the geometry and stability of this complex, and the way it allows assembly of Te atom dimers or oligomers. Reduction of Te(IV) by hydrazine was much slower than by the biomolecules and it is not dominant in early stages of the reduction process. This is proven by replacing hydrazine with non-reducing molecules containing amine groups that produce the same results (see Supplementary Fig. 6 ). Hydrazine addition before the reducing biomolecule caused a slower reduction by the biomolecule; hence, it was used to modify the kinetics of the reaction. Chiroptical properties Absorption and CD spectra of all the samples appear in Fig. 2 . As demonstrated in Fig. 2c , the CD could be reversed by choice of the opposite enantiomer of the biomolecule, indicating the formation of opposite crystal enantiomers. As the chiral biomolecules only absorb in the far ultraviolet region (<250 nm), the optical activity can only be assigned to excitation of states in the inorganic material. The intensity of chiroptical effects is usually evaluated by considering a normalized quantity, the dissymmetry factor, defined as the CD divided by absorption: . This eliminates concentration and extinction coefficient dependence when comparing different samples. 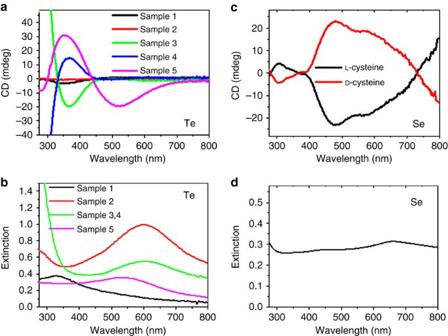Figure 2: CD and absorption spectra. CD and absorption spectra of tellurium (a,b) and selenium (c,d) samples. Tellurium sample 5 exhibits dissymmetry values much larger than for other samples of tellurium exceeding 0.003. For selenium,g-values exceed 0.002. Figure 2: CD and absorption spectra. CD and absorption spectra of tellurium ( a , b ) and selenium ( c , d ) samples. Tellurium sample 5 exhibits dissymmetry values much larger than for other samples of tellurium exceeding 0.003. For selenium, g -values exceed 0.002. Full size image For the Se nanocrystals, the extinction seemed to be dominated by scattering due to the relatively large size of the nanorods, and the peak dissymmetry value extracted from Fig. 2c,d was on the order of 0.002. Most of the Te samples had an observable CD peak in the near-ultraviolet region (~350 nm), indicating enantiomeric selectivity in the synthesis of the Te nanocrystals. Apart from the smallest particles in sample 1 ( Fig. 1a ), the other samples had strong extinction peaks at different wavelength in the visible range (between ~500 and 600 nm). However, only sample 5 ( Fig. 1e ) exhibited strong optical activity associated with its visible extinction peaks. Sample 2, in spite of strong visible extinction, exhibited weak CD activity across the near-ultraviolet–visible spectrum. There may be two possible explanations for this finding: First, at these specific conditions, enantiomeric excess achieved in the synthesis is small. Second, electronic transitions in Te across the visible spectrum are characterized by small Δ ε values. The second option is supported by the following results: the peak dissymmetry value of sample 5 exceeds 0.003, which is much larger than the other Te samples as well as most of past results on inorganic colloids. The intense chiroptical activity of sample 5 in comparison with other Te samples calls for consideration of an additional factor other than the chiral lattice symmetry: shape chirality. The shape of the particles from sample 5 was characterized using scanning TEM (STEM) tomography. 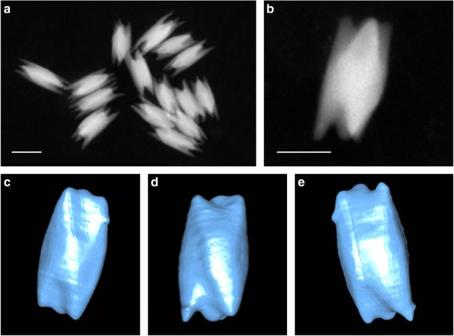Figure 3: Dark-field STEM imaging and tomography of tellurium sample 5. (a,b) STEM images at two magnifications. (c–e) Tomographic reconstruction of the particle inb, as observed from three different orientations. Chirality is observed in the twisted ridges crossing diagonally between vertices at the two ends, always stretching from bottom right to top left. Scale bars, 100 nm. Electron tomography Figure 3a,b depict these particles as observed in STEM mode with a dark-field detector. Figure 3c–e display snapshots from the three-dimensional (3D) tomographic reconstruction at different orientations (see also Supplementary Movie 1 ) of the particle in Fig. 3b . The basic shape of the nanoparticles is approximately trigonal prism. The handedness of each particle can be determined when observing the side faces, where there are twisted ridges crossing diagonally between vertices at the two opposite ends of the prisms. Figure 3: Dark-field STEM imaging and tomography of tellurium sample 5. ( a , b ) STEM images at two magnifications. ( c – e ) Tomographic reconstruction of the particle in b , as observed from three different orientations. Chirality is observed in the twisted ridges crossing diagonally between vertices at the two ends, always stretching from bottom right to top left. Scale bars, 100 nm. Full size image Nanocrystals obtained with D -glutathione exhibited similar but more deformed shapes, as well as the opposite handedness and CD with a smaller magnitude and slightly different lineshape (see Supplementary Fig. 7 ). The inexact mirror image CD lineshape and particle shape are due to the lower purity of the D- form of glutathione (nominally 95%) that was obtained synthetically, relative to L -glutathione (98%). In contrast to this, all samples prepared with penicillamine or cysteine (for which both enantiomers are available commercially at same levels of purity) showed an exact mirror image CD behaviour for opposite enantiomers. Evolution of Te nanostructures with chiral shape The mechanism of growth of these shapes was examined in a series of syntheses and TEM experiments, where the growth of these structures was arrested at various stages of the evolution of the trigonal shapes. The reaction was quenched at each interval by mixing a fraction that is removed from the synthesis with a concentrated solution of SDS at room temperature (1:1 volume ratio of sample and 100 mM SDS solution). As shown in Fig. 4a (and Supplementary Fig. 8 ), these nanostructures seem to be forming by coalescence of small clusters. The smaller shapes shown in Fig. 4a (developed after 2 min of reaction) had an average length of 70±20 nm. The particles of sample 5 (15 min reaction) were the next intermediate stage observed ( Figs 1e and 4b ). These particles had an average length of 140±25 nm. These further grew to ~200-nm-long hexagonal tubes depicted in Fig. 4c (20 min). After reacting for 1 h, longer tubes of ~300 nm and different morphology were obtained ( Fig. 4d ). The trigonal and hexagonal cross sections evolving in this process are well observed for particles in dense samples that agglomerate and orient perpendicular to the carbon support film ( Fig. 4e,f —corresponding to the samples shown in Fig. 4a,c ). 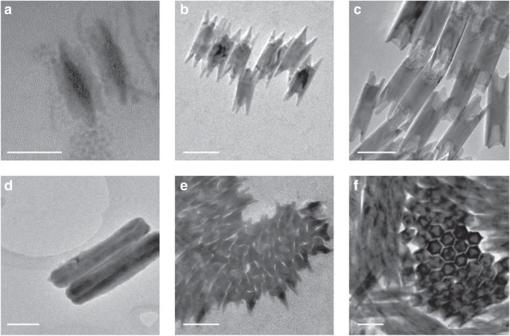Figure 4: TEM images of nanocrystals of sample 5 showing evolution over time. (a) Small nanocrystals are initially formed with very small clusters added to the structure. Scale bar, 50 nm. (b) Larger nanocrystals are viewed after another 13 min of reaction. Scale bar, 100 nm. (c) These evolve into fractured hexagonal tubes. Scale bar, 100 nm. (d) Eventually long hollow tubes are formed. Scale bar, 100 nm. (e,f) Images of nanocrystals from the same samples as inaandc, respectively, when arranged with the long axis perpendicular to the surface in dense arrays. Scale bar, 100 nm. The transition from trigonal to hexagonal cross section is observed. Figure 4: TEM images of nanocrystals of sample 5 showing evolution over time. ( a ) Small nanocrystals are initially formed with very small clusters added to the structure. Scale bar, 50 nm. ( b ) Larger nanocrystals are viewed after another 13 min of reaction. Scale bar, 100 nm. ( c ) These evolve into fractured hexagonal tubes. Scale bar, 100 nm. ( d ) Eventually long hollow tubes are formed. Scale bar, 100 nm. ( e , f ) Images of nanocrystals from the same samples as in a and c , respectively, when arranged with the long axis perpendicular to the surface in dense arrays. Scale bar, 100 nm. The transition from trigonal to hexagonal cross section is observed. Full size image The self-assembly process that is observed at the initial stages of this reaction is intriguing. Recently, Viedma et al . [34] reported a mechanism for growth of chiral crystals through ‘enantiomer-specific oriented attachment’. It seems that in the Te structures presented here, such a process is taking place at the nanoscale, where initially formed chiral atomic clusters attach in an oriented way to form a chiral nanocrystal. It can be seen that the shapes of the evolving Te nanostructures are generally quite complex. The sensitivity of the shape to the particular structure of the chiral thiolated surfactant molecules further strengthens the hypothesis of growth by oriented attachment of surfactant-coated atomic clusters. However, it is still a puzzle how these local attachment effects would lead to shape chirality on a larger (10–100 nm) scale. Local strain effects caused by the chiral surfactant packing at the surface might be responsible for chiral shape distortions. 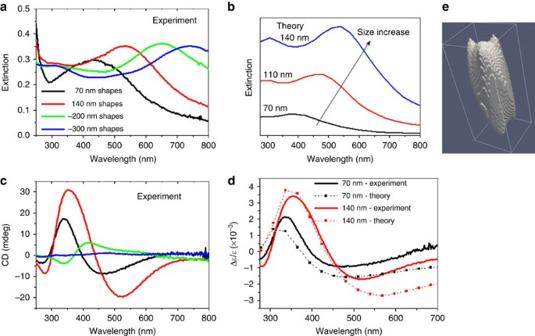Figure 5: Absorption and CD activity of chiral shapes of tellurium. Experimental (a) and simulation (b) absorption spectra of samples displayed inFig. 4. Red shift of the peak position with size is observed. (c) Experimental CD of samples. (d) Experimental and simulated dissymmetry spectra for two different size samples. (e) Model chiral shape used in the simulation. Figure 5 displays the absorption and CD spectra of aqueous dispersions of the series of chiral shapes shown in Fig. 4 . The first interesting observation, seen in Fig. 5a , is of a red shift between 450–750 nm in the major absorption/extinction feature with increase in particle dimension (see also Supplementary Fig. 9 ). Figure 5: Absorption and CD activity of chiral shapes of tellurium. Experimental ( a ) and simulation ( b ) absorption spectra of samples displayed in Fig. 4 . Red shift of the peak position with size is observed. ( c ) Experimental CD of samples. ( d ) Experimental and simulated dissymmetry spectra for two different size samples. ( e ) Model chiral shape used in the simulation. Full size image Model electromagnetic calculations As seen in Fig. 5b , the spectral shift is reproduced by a discrete dipole approximation (DDA) calculation [35] of the extinction using the bulk Te dielectric constant [36] . The DDA method is very convenient for computational studies of CD signals,as it permits calculations of extinction with a very high precision. For our goal, we need a high precision, as CD signals are typically much weaker than extinction coefficients. In a recent publication, Fan et al . [37] have demonstrated that the DDA method is suitable for calculations of weak chiroptical signals of plasmonic nanostructures. The shape of the particle used in the model was similar to the experimental shapes obtained from the tomogram and the dimensions of the model shape were adjusted according to the TEM measurements. The shift in extinction spectra with size is due to length-dependent electromagnetic resonance modes of these shapes. As Te exhibits a continuum of absorbing states throughout the near-ultraviolet–visible–near-infrared range, those electromagnetic resonances enhance the extinction of the nanoparticles at the resonance wavelengths. In addition, an absorption peak at 300–350 nm, which does not shift with shape or size change, is observable for the larger nanostructures (where there is no spectral overlap with the electromagnetic resonance mode), both in the experimental and simulated absorption spectra of Fig. 5a,b . Thus, it seems that the near-ultraviolet transition around 300–350 nm is associated with localized Te states and carries a weak CD signal, which is related to the chiral atomic configuration. The CD spectra of the chiral particle series displayed in Fig. 5c shows that the CD lines also shift with size as observed with the absorption spectra. The DDA simulated CD dissymmetry factor spectra for two different sizes, plotted in Fig. 5d together with experimental dissymmetry spectra of nanostructures of similar sizes, are only based on the shape chirality and ignore the atomic scale chirality. Considering the rough approximation of shape and size, the simulated spectra agree well with the experimental dissymmetry factors both in wavelength and intensity. The fit between the single particle (100% enantiomeric excess) simulated CD amplitude and experimental CD amplitude serves as an indication that at least for sample 5, the enantiomeric excess is high, although it is not yet possible to give an exact value. For nanocrystals with chiral lattice and an achiral shape, estimation of enantiomeric excess is currently an unresolved challenge. For the earlier case of α-HgS [28] , where data from bulk was available regarding CD strength, the enantiomeric purity was estimated to be very high under similar synthetic conditions as the current work. However, it is not clear that all materials will yield similar enantioselectivity in the synthesis, and future development of a method to determine enantiomeric excess in these systems, in a more general and exact way, would be indispensable. The optical response of the Te nanostructures is quite unique relative to other colloidal nanomaterials. Although in wide gap semiconductors there are quantum size effects governing the spectral shifts (for sizes of several nanometres), in the present case the relatively large size of the nanostructures rules out such effects, and as the DDA simulation confirms the size effects come from enhancement of absorption at wavelengths where electromagnetic cavity resonance modes occur. This, together with the shape chirality, turn the Te nanostructures shown in Figs 3 and 4 into a unique case of nanoscale chiral optical resonators. The CD activity of the Te nanocrystals, observed both experimentally and theoretically, is due to the chiral shape of an absorbing and scattering object made of a semiconductor ( Supplementary Fig. 10 ). This mechanism is somewhat different from the mechanisms leading to CD in molecules [38] , [39] and also different from the case of metal nanostructures [5] , [6] , [7] , [8] . In metal nanostructures the CD has a plasmonic origin, whereas in Te nanocrystals the CD originates from inter-band exciton transitions as well as scattering of the large dielectric nanonanostructures with chiral shapes. Another finding out of the simulations is that the bisignate CD spectrum of a Te twister is relatively insensitive to its shape. Different right-handed shapes of a twister with the same overall size were simulated and always yielded CD spectra with positive short-wavelength part and a negative long-wavelength region (see Supplementary Fig. 11 ). Transformation of chiral Te nanostructures into other materials The reactivity of elemental Te to chemical transformations holds promise for templating of chiral nanostructures of various materials by depositing them on the chiral Te nanostructures. Here we demonstrate templating of chiral gold and silver telluride nanostructures. Many reports, such as by Sanchez-Iglesias et al . [40] , demonstrate templating of plasmonic gold particles by galvanic replacement of Te nanocrystals. Transformation of Te nanostructures to silver telluride can also be achieved easily by reaction with silver ions [41] . When nanocrystals of sample 5 were used as sacrificial templates, gold and silver telluride nanostructures with unique shapes were formed. TEM images of these particles together with their extinction and CD spectra are presented in Fig. 6 (see also material characterizations in Supplementary Figs 12–14 ). These transformations preserve the chiral shape very efficiently. For the gold nanostructures, an exceptionally large plasmonic CD with peak dissymmetry around 650 nm of ~0.015 was obtained. The two peaks seen in the absorption spectrum of this sample are the typical transverse (~550 nm) and longitudinal (~900 nm) resonances observed in elongated gold nanostructures. Thus, we see that the CD peak extending from 600 nm onward into the infrared corresponds to the longitudinal plasmonic resonance, which is apparently more sensitive to the twist in the nanostructure than the transverse resonance. At the wavelength of the transverse resonance there is no noticeable CD signal. We may expect this, as the transverse plasmons create typically less absorption and exhibit much weaker CD. 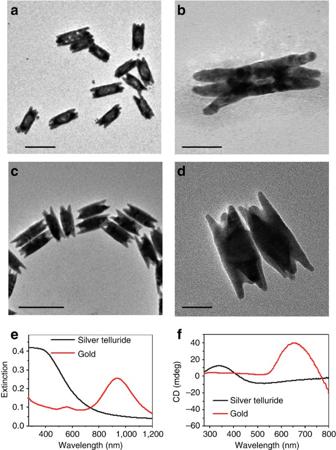Figure 6: Nanocrystals of gold and silver telluride formed by chemical transformation. (a,b) TEM images of such gold nanostructures. (c,d) TEM images of silver telluride nanocrystals. (e) Extinction and (f) CD spectra are depicted in the bottom row. Scale bars, 200 nm (a,c) and 50 nm (b,d). Figure 6: Nanocrystals of gold and silver telluride formed by chemical transformation. ( a , b ) TEM images of such gold nanostructures. ( c , d ) TEM images of silver telluride nanocrystals. ( e ) Extinction and ( f ) CD spectra are depicted in the bottom row. Scale bars, 200 nm ( a , c ) and 50 nm ( b , d ). Full size image Colloidal nanostructures of Se and Te with various morphologies and large enantiomeric excess were prepared with the use of strongly binding chiral ligands and the extinction and CD spectra analysed. For Se samples, the CD is assigned to the intrinsic chirality of the crystal structure and the enantiomeric excess of nanocrystals formed in the synthesis. For Te, two hierarchies of chirality have been observed. For chiral lattice and achiral shape (nanorods), the dissymmetry value is small. For the case of chiral lattice and chiral shape (sample 5), the peak dissymmetry was very large. These observations were correlated with electromagnetic response simulations to prove that for Te the shape chirality is much more significant for visible wavelengths chiroptical activity than lattice chirality. Thus, the chiral Te nanostructures of size of the order of 100 nm act as chiral optical resonators, and might become useful in optical sensing of chiral molecules. The results presented in this work prove that the concept of enantioselective synthesis of intrinsically chiral inorganic nanocrystals could be generalized to many material systems. A wide variety of chiral inorganic materials still remain for future studies, such as different crystals of SiO 2 and GeO 2 , AlPO 4 , Ag 2 Se, CrSi 2 , HgO, TeO 2 and more. Control over chirality in these systems may sometimes be not limited to lattice symmetry and may extend to the shape of the whole particle, making these systems intriguing for studies of chirality-associated effects at several size hierarchies. In this regard, the present work gives a first demonstration of mesoscale shape chirality for Te. Relation of shape to molecular scale chirality has been considered in the formation of chiral (twisted) mesoscopic shapes in several material systems [42] , [43] , [44] . For inorganic crystals, this has been observed in bulk form, in quartz for instance [45] . However, the exact mechanism of translation of molecular scale lattice chirality into whole crystal shape chirality is not fully established. We believe that the kind of material systems studied here are excellent candidates to test the generality of this concept and address the mechanisms involved. It is expected that intrinsically chiral materials should be very useful for enantioselective chemistry (for which the lattice chirality is sufficient), as recently demonstrated by Soai and colleagues [46] for asymmetric autocatalysis induced by macroscopic α-HgS crystals. Nanocrystals should be even more efficient as catalysts due to much higher surface-to-volume ratio. In addition, recent reports indicate that materials composed of helical morphologies should be useful for spintronics applications [47] . On a fundamental level, these systems are expected to be intriguing candidates for studies of mechanisms acting in chiral crystallization, as well as studies of binding of organic molecules to chiral surfaces [1] , [2] , which is a key aspect in catalysis. An advantage of such studies is that the nano-colloidal systems are easy to monitor spectroscopically, as opposed to bulk solid-state samples where chiroptical spectroscopy is challenging [48] . One important message from this work is that although chiral crystals have been considered as sources for generation of homochirlity in biomolecules, the opposite effect of biomolecules inducing homochirality in crystals is also fascinating. The reactivity of Te towards chemical transformations might aid in future design of chiral nanostructure shapes of achiral materials, such as presented here for gold and silver telluride. Specifically, for the case of metallic systems with plasmon resonances, this method could be further developed for large-scale production of chiral meta-materials. Chemicals Tellurium dioxide (TeO 2 ; 99.995%), selenous acid (98%), gold chloride trihydrate (≥99.9%), silver nitrate (99.9%), hydrazine hydrate solution (78–82%), L -glutathione (reduced form, ≥98% ), L -cysteine (≥98.5%), D -cysteine (≥99%), L -penicillamine (99%), D -penicillamine (≥99%), L -arginine (≥98%), SDS (99%), sodium borohydride (98%) and sodium hydroxide (97%) were purchased from Sigma and used without further purification. D -glutathione (purity according to HPLC 95%) was obtained from Genscript USA, Inc. All water used was ultrapure (18 MΩ cm), obtained from a USF ELGA UHQ system Synthesis For the biomolecule stock solutions, the reagent (glutathione, cysteine, penicillamine) was dissolved in water (final concentration 100 mM). Afterwards, the pH was adjusted to 11.5 using NaOH solution (1 M). For the TeO 2 solution, 15 mg of TeO 2 was dispersed in 1 ml of 20 mM NaOH aqueous solution. The material is only slightly soluble, and the solution remained turbid and was constantly stirred before and during the reaction. All samples were prepared in 20 ml glass vials, placed on a hot plate with magnetic stirring. To stop the reaction, 1 ml of the sample was collected and diluted twice with 100 mM SDS solution in water at room temperature. Te nanocrystals (1) The temperature of the plate was set to 62 °C. The following reagents have been added in this order: 1 ml TeO 2 solution, 1 ml L -glutathione solution and 8 ml water. The sample was collected after 10 min reaction. Te nanorods (2) The temperature of the plate was set to 62 °C. The following reagents were added in this order: 1 ml TeO 2 solution, 1 ml L -glutathione solution and 5.5 ml water were added (fast), followed by dropwise addition of 2.5 ml hydrazine solution. Aliquots of the reaction have been removed every 10 min. Te nanocrystals (3 and 4) The temperature of the plate was set to 62 °C. The following reagents were added in this order: 1 ml TeO 2 solution, 1 ml L - or D - penicillamine solution and 5.5 ml water were added (fast), followed by dropwise addition of 2.5 ml hydrazine solution. The sample was obtained after 30 min of reaction. Te nanocrystals (5) The following reagents were added in this order: 1 ml TeO 2 solution, followed by 5.5 ml water and dropwise addition of 2.5 ml hydrazine solution. Finally 1 ml glutathione ( L - or D -form) solution was added. Aliquots were collected at different time intervals as described in the main text. Se nanocrystals To 2 ml of water, 0.1 ml aqueous solution of selenous acid (100 mM) was added, followed by 0.1 ml of hydrazine hydrate solution. After that, the pH was raised by addition of 0.02 ml NaOH solution (1 M), and finally 0.1 ml cysteine solution ( L - or D- form, 100 mM in water) was added. The reaction was left for 24 h at room temperature in the dark. During that time the colour gradually evolved from yellow to orange to pink/purple. After that, the particles were collected by centrifugation and washed with water several times, followed by addition of 100 mM SDS for stabilization. Conversion of chiral Te nanostructures to gold Sample 5 (0.5 ml; diluted × 2 with 100 mM SDS solution) was purified by collecting the particles sediment after centrifugation, removing all the solution and dispersing in water (several times). After that, the particles were finally dissolved in 2 ml water. A gold precursor solution containing 1 ml of 100 mM CTAB solution, 0.2 ml HAuCl 4 solution and 0.1 ml NaOH (1 M) solution was prepared. Of this solution, a quantity of 0.4 ml was added to 2 ml of purified sample 5 particles, and the reaction was left for 1 h before collecting the particles by centrifugation and washing with water several times. Conversion of chiral Te nanostructures to silver telluride Sample 5 (diluted × 2 with 100 mM SDS solution) was cleaned as described in the procedure of gold templating. Of the clean sample, 0.5 ml were diluted with 1.5 ml water and stirred vigorously. AgNO 3 solution (0.06 ml) in water (100 mM) was added, and the solution was left to react for 1 h. After that, particles were collected and cleaned by centrifugation. Spectroscopic and structural characterization CD measurements were performed using an Applied Photophysics Chirascan spectrometer. Absorption measurements were performed using a Varian Carry 5000 spectrophotometer. TEM imaging and diffraction was performed using a FEI Tecnai F20 FEG-TEM, with a gold nanoparticle standard used for calibration in diffraction. STEM imaging and tomography, as well as energy dispersive X-ray spectroscopy measurements, were performed using a Tecnai F-20 S/TEM microscope (Twin lens) equipped with a Fischione Model 3000 high-angle annular dark-field detector. Electron tomography Tomographic data sets were obtained using Xplore3D software (FEI). Images were acquired in a tilt range of ±70°, with a ° increment at the lower tilts (less than 46° tilt) and a 1° increment at the higher tilts. In total, 94 images were acquired. The images were aligned and reconstructed using a refinement procedure for the image alignment, which uses an iterative optimization of the tomogram resolution and SIRT algorithm for the subsequent tomogram reconstruction [49] . Three-dimensional visualization was performed by ImageVis3D freeware, version 3.0.0, developed at the University of Utah. DDA calculations and model The computational results given in the manuscript are based on a numerical solution of Maxwell’s equations incorporating local dielectric functions of Te [36] and water as a medium. ( ε water =1.8) The Te crystal has intensive inter-band transitions that are reflected in the real and imaginary parts of the dielectric constant [36] . As a numerical method, we employed the DDA [35] , [50] and the software from http://www.astro.princeton.edu/~draine/DDSCAT.html and ref. 51 . CD is calculated as a difference of the optical extinctions for left and right circularly polarized (LCP and RCP) light beams: Δ ε = ε LCP − ε RCP , where ε LCP and ε RCP are the extinction coefficients for the corresponding circularly polarized photons. Note that, in our calculations, the above extinction coefficients were averaged over the orientation of a nanocrystal relative to the direction of incident light [52] . To mimic the Te nanocrystals synthesized in the project, we tried several shapes. The shape, which most closely resembles the experimental nanoparticles ( Fig. 3 ), is shown in Fig. 5e . This shape is made of four merged nanorods. One wide nanorod is placed in the centre of the construction and the other three nanorods are attached to the central one. In addition, we created twisted stripes on the sides of the object and these stripes brought chirality to this geometry. In the first step, we created a mathematical function in the spherical coordinates, ρ = f ( θ , ϕ ), that defines the surface of such particle ( Supplementary Fig. 10 , inset). In the next step, we filled this geometrical object with point dipoles ( Supplementary Fig. 15 , inset). This is the model for the DDA computation. Within the DDA approach, a crystalline object is represented as a set of point dipoles with certain polarizability and density values. When the number of dipoles is very large, the DDA model is reliable and describes very well optical properties of the initially continuous object. Here we apply this method for semiconductor nanocrystals with strong absorption and scattering. Supplementary Fig. 15 shows the reliability of our calculations. As an example, we consider the Te twister with the 140-nm length. We now vary the number of point dipoles in the DDA calculations, denoted as N dipoles , by ~8 times and we do not observe significant changes in the calculated CD spectra. Our calculation results shown in Fig. 5b,d and Supplementary Fig. 10 were done for N dipoles =1.5 × 10 5 , whereas Supplementary Fig. 15 depicts the data for three numbers N dipoles =6.5 × 10 4 , 1.5 × 10 5 and 5.1 × 10 5 . How to cite this article: Ben-Moshe, A. et al . Enantioselective control of lattice and shape chirality in inorganic nanostructures using chiral biomolecules. Nat. Commun. 5:4302 doi: 10.1038/ncomms5302 (2014).